Differentiation-dependent requirement of Tsix long non-coding RNA in imprinted X-chromosome inactivation Imprinted X-inactivation is a paradigm of mammalian transgenerational epigenetic regulation resulting in silencing of genes on the paternally inherited X-chromosome. The preprogrammed fate of the X-chromosomes is thought to be controlled in cis by the parent-of-origin-specific expression of two opposing long non-coding RNAs, Tsix and Xist, in mice. Exclusive expression of Tsix from the maternal-X has implicated it as the instrument through which the maternal germline prevents inactivation of the maternal-X in the offspring. Here, we show that Tsix is dispensable for inhibiting Xist and X-inactivation in the early embryo and in cultured stem cells of extra-embryonic lineages. Tsix is instead required to prevent Xist expression as trophectodermal progenitor cells differentiate. Despite induction of wild-type Xist RNA and accumulation of histone H3-K27me3, many Tsix-mutant X-chromosomes fail to undergo ectopic X-inactivation. We propose a novel model of lncRNA function in imprinted X-inactivation that may also apply to other genomically imprinted loci. X-chromosome inactivation results in the mitotically stable epigenetic transcriptional silencing of genes along one of the two X-chromosomes in female mammals, thereby equalizing X-linked gene expression between males and females [1] . X-inactivation is thought to be separable into three phases: initiation, establishment and maintenance [2] . During the initiation phase, cell autonomous epigenetic mechanisms identify the future inactive X-chromosome and trigger the formation of transcriptionally inert heterochromatin on that X. This heterochromatic configuration is then proposed to spread during the establishment phase to envelop genes across most of the inactive X-elect. Once inactivated, replicated copies of that X-chromosome are transmitted as inactive through multiple cell division cycles during the maintenance phase. While one X-chromosome is transmitted as inactive during mitosis, the other X within the same nucleus is maintained in a transcriptionally active state. The epigenetic transcriptional states of both the inactive and active X-chromosomes are controlled in cis by a segment on the X-chromosome that encodes long non-coding RNAs (lncRNAs), which play key roles in both X-inactivation and in forestalling inactivation of the active-X [3] , [4] , [5] . The two most prominent lncRNAs are Xist and Tsix. Xist is induced exclusively from the inactive X-chromosome and is considered a primary determinant of X-inactivation [6] , [7] . Current models posit that Xist RNA transcription initiates a cascade of events that ultimately leads to X-inactivation [8] . Xist RNA physically coats the chromosome from which it is expressed, leading to the deposition of proteins that catalyse epigenetic transcriptional silencing along this X-chromosome [9] . The most notable of the Xist RNA recruits are Polycomb group proteins. Distinct Polycomb group complexes are thought to contribute to the formation of the unique facultative heterochromatic structure of the inactive-X via post-translational modification of histones [10] , [11] , [12] , [13] . While expression of the Xist RNA is required in cis for X-inactivation, transcription of the Xist anti-sense RNA, Tsix, is necessary to prevent inactivation of the active-X [14] , [15] , [16] . Tsix transcription across the Xist gene is posited to inhibit Xist expression, potentially by influencing chromatin modifications at the Xist promoter [17] , [18] . In mice, all cells of the developing zygote initially undergo imprinted inactivation of the paternal X-chromosome, beginning at around the 4–8 cell stage of zygotic development [19] , [20] , [21] , [22] . The preprogrammed fate of the two Xs during imprinted X-inactivation implies that the X-chromosomes are differentially marked in the parental germlines. In the preimplantation embryo, Xist is expressed exclusively from the paternal-X and Tsix only from the maternal-X [15] , [16] . The mutually exclusive expression and divergent transcriptional impact of Xist and Tsix lncRNAs represent a paradigm of how parent-of-origin-specific gene regulation is executed in the offspring [23] . While the paternal-X undergoes imprinted X-inactivation, evidence indicates that the epigenetic imprint itself resides on the maternal-X [24] . This notion is supported by the observation that in early embryos that harbour two maternal X-chromosomes, neither X-chromosome undergoes X-inactivation [25] , [26] , [27] . Conversely, embryos with two paternal-Xs initially express Xist from both X-chromosomes, but then downregulate Xist from one of the two Xs and appear to stably inactivate the other Xist-coated X-chromosome [28] . Due to its expression exclusively from the maternal-X, its Xist -antagonistic function, and that embryos harbouring a Tsix-mutant maternal X-chromosome die during gestation, Tsix RNA has been nominated as the factor via which the oocyte prevents inactivation of the maternal X-chromosome in the embryo [15] , [16] . However, the temporal requirement of Tsix in imprinted X-inactivation, that is, whether it functions during the initiation phase in the early embryo, which would support an oogenic imprint role, or in the maintenance phase in the later embryo, remains unclear. At the peri-implantation (~128-cell) stage of embryogenesis, the pluripotent epiblast precursor cells in the inner cell mass (ICM) compartment reactivate the inactive paternal X-chromosome [29] , [30] . The epiblast lineage is the sole contributor of cells that will form the fetus; the rest of the cells from the early embryo give rise to the trophectoderm and the primitive endoderm lineages that will contribute to the extra-embryonic structures of the placenta and yolk sac, respectively [31] . After the embryo implants, descendants of the epiblast precursor cells undergo transcriptional reactivation of the paternal X-chromosome, followed by random X-inactivation of either the maternal or paternal X-chromosome [32] . The transcriptional reactivation of the inactive paternal X-chromosome in pluripotent epiblast progenitors is characterized by loss of Xist RNA coating [29] , [30] , [33] . Xist RNA depletion is thought to contribute to the epigenetic remodelling of the inactive paternal X-chromosome, leading to the re-expression of paternal X-linked genes [29] . Similarly, Xist repression and the absence of or reactivation of the inactive-X are considered epigenetic hallmarks of pluripotency; female mouse embryonic stem (ES) cells and induced pluripotent stem cells both display two active-Xs [34] , [35] , [36] . As a negative regulator of Xist, Tsix is proposed to facilitate the loss of Xist RNA coating and reactivation of the inactive-X [37] , [38] , [39] . To date, however, genetic evidence linking Tsix expression to Xist repression during X-chromosome reactivation is lacking. Here, we comprehensively examine the role of Tsix RNA in imprinted X-inactivation and -reactivation in vivo and in vitro . We find that Tsix is dispensable in suppressing Xist and for preventing X-inactivation during the initiation as well as maintenance phases of imprinted X-inactivation through studies in the preimplantation embryo and in stem cells of the trophectoderm and primitive endoderm lineages. Instead, Tsix is required to prevent Xist induction during the differentiation of trophoblast cells in vivo an in vitro . Despite the induction of intact Xist RNA and accumulation of Polycomb group-catalysed histone methylation on the Tsix-mutant X-chromosome, a substantial number of trophoblast cells do not display ectopic X-inactivation. We further find that both the repression of Xist and the reversal of imprinted X-inactivation that occur in epiblast precursor cells prior to random X-inactivation do not require Tsix RNA. Role of Tsix during initiation of imprinted X-inactivation If Tsix expression serves to repress Xist during the initiation phase of imprinted X-inactivation, then a maternal-X devoid of Tsix RNA should ectopically express Xist in the preimplantation embryo. We therefore generated embryonic day (E) 3.5 blastocyst-stage (~64-cell) embryos that inherit either a wild-type (WT) or a Tsix-mutant maternal-X from Tsix heterozygous females. The Tsix mutation, Tsix AA2Δ1.7 , truncates the Tsix transcript in exon 2 and deletes the critical DXPas34 repeat sequence that controls Tsix expression (herein referred to as X ΔTsix ) ( Fig. 1a ) [16] , [40] , [41] , [42] . Since Tsix transcription across the Xist promoter region is required for Tsix RNA to inhibit Xist expression, X ΔTsix is functionally a null Tsix mutation [16] , [17] , [18] . We first assayed Tsix and Xist expression by RNA fluorescence in situ hybridization (RNA FISH) with single-stranded riboprobes that uniquely detect Tsix or Xist. Tsix expression is detectable from the active (maternal) X-chromosome in most nuclei of approximately half of the embryos; in the remaining embryos, Tsix is undetectable in all nuclei ( Fig. 1b ). The active-X is additionally marked by expression of the Atrx gene, which is subject to X-inactivation. We therefore classified embryos with Tsix RNA FISH signals as WT XX and XY and the ones without as mutant X ΔTsix X and X ΔTsix Y . These embryos displayed Xist RNA coating in XX but not XY embryos, as expected ( Fig. 1b ). To our surprise, X ΔTsix X blastocysts also showed Xist RNA coating of only one X-chromosome, and lack of inactivation of the X ΔTsix maternal X-chromosome ( Fig. 1b,c ). As in X ΔTsix X females, X ΔTsix Y males also failed to display Xist induction or defective gene expression from their single, maternally inherited X-chromosome ( Fig. 1b,c ). 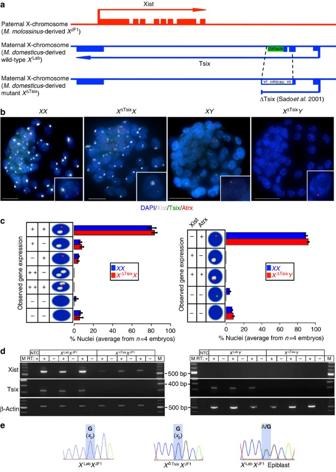Figure 1: Absence of ectopic Xist induction from theXΔTsixmaternal X-chromosome in embryonic day (E) 3.5 blastocyst embryos. (a) Schematic representation of the genomic structure ofXist,Tsixand the Tsix RNA truncation-mutantXΔTsix. (b) RNA FISH detection of Xist (white), Tsix (green) and Atrx (red) RNAs in representative E3.5 embryos. Nuclei are stained blue with 4′,6-diamidino-2-phenylindoledichloride (DAPI). Insets show representative nuclei. Scale bar, 25 μm. (c) Quantification of Xist, Tsix and Atrx RNA expression patterns in blastocyst nuclei. Thexaxis of each graph represents the average % nuclei observed in each class for each genotype.n=4 embryos per genotype. Diagrams along theyaxis depict all observed expression patterns. +, RNA expression detected from a single X-chromosome; ++, RNA expression detected from both X-chromosomes; −, absence of RNA detection. Gene expression patterns do not differ significantly between WT and Tsix-mutant blastocysts (Fisher’s exact test). Error bars, s.d. (d) RT–PCR detection of Xist, Tsix and control β-actin RNAs. Three individual embryos are shown for each genotype. M, marker; NTC, no template control; +, reaction with reverse transcriptase (RT); −, no RT control lane. (e) Sanger sequencing chromatograms of representative Xist RT–PCR products. Highlights mark a single nucleotide polymorphism that differs between the maternalXLab/XΔTsixalleles and the paternalXJF1allele (see Methods). BothXLabXJF1andXΔTsixXJF1females express Xist only from the paternally inherited X-chromosome (Xp). TheXLabXJF1epiblast is a control sample displaying expression from both parental alleles. Figure 1: Absence of ectopic Xist induction from the X ΔTsix maternal X-chromosome in embryonic day (E) 3.5 blastocyst embryos. ( a ) Schematic representation of the genomic structure of Xist , Tsix and the Tsix RNA truncation-mutant X ΔTsix . ( b ) RNA FISH detection of Xist (white), Tsix (green) and Atrx (red) RNAs in representative E3.5 embryos. Nuclei are stained blue with 4′,6-diamidino-2-phenylindoledichloride (DAPI). Insets show representative nuclei. Scale bar, 25 μm. ( c ) Quantification of Xist, Tsix and Atrx RNA expression patterns in blastocyst nuclei. The x axis of each graph represents the average % nuclei observed in each class for each genotype. n= 4 embryos per genotype. Diagrams along the y axis depict all observed expression patterns. +, RNA expression detected from a single X-chromosome; ++, RNA expression detected from both X-chromosomes; −, absence of RNA detection. Gene expression patterns do not differ significantly between WT and Tsix-mutant blastocysts (Fisher’s exact test). Error bars, s.d. ( d ) RT–PCR detection of Xist, Tsix and control β-actin RNAs. Three individual embryos are shown for each genotype. M, marker; NTC, no template control; +, reaction with reverse transcriptase (RT); −, no RT control lane. ( e ) Sanger sequencing chromatograms of representative Xist RT–PCR products. Highlights mark a single nucleotide polymorphism that differs between the maternal X Lab / X ΔTsix alleles and the paternal X JF1 allele (see Methods). Both X Lab X JF1 and X ΔTsix X JF1 females express Xist only from the paternally inherited X-chromosome ( X p). The X Lab X JF1 epiblast is a control sample displaying expression from both parental alleles. Full size image To independently validate the RNA FISH data, we performed allele-specific RT–PCR amplification of Xist RNA in individual F1 hybrid blastocyst-stage embryos harbouring polymorphic X-chromosomes. While the maternal X-chromosome is transmitted by M. domesticus- derived laboratory and Tsix-mutant strains (WT X Lab and mutant X ΔTsix , respectively), the paternal X-chromosome is derived from the divergent M. molossinus JF1 ( X JF1 ) strain; these strains contain numerous single nucleotide polymorphisms (SNPs), which permits defining the allele-specific origin of RNAs. We again assigned genotypes to the embryos by assaying Tsix RNA expression ( Fig. 1d ). As expected, in WT X Lab X JF1 and X Lab Y , embryos Xist was expressed only in females and not in males ( Fig. 1d ). We observed a similar pattern of Xist RNA expression in X ΔTsix X JF1 and X ΔTsix Y mutant blastocysts ( Fig. 1d ). X ΔTsix Y -mutant males did not exhibit Xist expression, consistent with the RNA FISH data. We exploited a SNP in the Xist RT–PCR amplicon to identify the chromosomal source of Xist RNA in X Lab X JF1 and X ΔTsix X JF1 embryos. Both genotypes displayed Xist expression only from the paternal X-chromosome ( Fig. 1e ). Taken together, the RNA FISH and RT–PCR results lead us to conclude that Tsix is dispensable in preimplantation embryos during the initiation phase of imprinted X-inactivation, both to prevent Xist expression and to forestall inactivation of the maternally inherited X-chromosome. Post-implantation role of Tsix in suppressing Xist Maternally inherited Tsix mutations are typically embryonic lethal, suggesting an essential requirement for Tsix during embryonic development [15] , [16] . Since X ΔTsix X and X ΔTsix Y preimplantation embryos displayed normal imprinted X-inactivation, we investigated imprinted X-inactivation in peri- and post-implantation embryos to pinpoint when Tsix is required. At the E4.0 peri-implantation stage, X ΔTsix X and X ΔTsix Y embryos begin to exhibit Xist induction from the X ΔTsix X-chromosome in a few nuclei, typically fewer than 3% ( Supplementary Fig. 1 ). We next examined Xist expression and X-inactivation in XX , X ΔTsix X , XY and X ΔTsix Y E6.5 post-implantation embryos. We initially assessed Xist RNA coating and expression of the X-linked gene Pgk1 , which is subject to X-inactivation, in whole E6.5 embryos using double-stranded probes that detect Xist and Tsix simultaneously [21] , [43] . At E6.5, the extra-embryonic cell types derived from the trophectoderm and the primitive endoderm of earlier embryos normally maintain imprinted X-inactivation, while the epiblast cells display random X-inactivation. We observed ectopic Xist expression from the mutant X-chromosome in both X ΔTsix X and X ΔTsix Y embryos but not in WT XX and XY counterparts ( Supplementary Fig. 2a–d , Supplementary Movies 1–4 ). Using single-stranded riboprobes, we next quantified Xist RNA coating and Pgk1 expression in isolated extra-embryonic tissues and found that 15% of X ΔTsix X and 12% of X ΔTsix Y cells showed ectopic Xist RNA coating and Pgk1 silencing. These percentages represent a significant level of ectopic X-inactivation in extra-embryonic cells ( P= 3.5 × 10 −5 and P =0.0003, respectively, Fisher’s exact test; Fig. 2a,b ). We confirmed ectopic expression of Xist RNA from the maternal X-chromosome in mutant extra-embryonic cells and its absence in WT cells by allele-specific RT–PCR followed by Sanger sequencing to determine the allelic origin of the transcript ( Fig. 2c,d ). Tsix deficiency, therefore, induces Xist expression and inactivation of the maternal X-chromosome in the extra-embryonic tissues of post-implantation embryos. 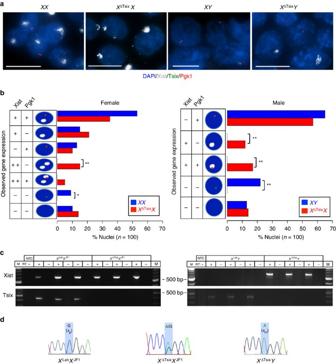Figure 2: Xist induction from theXΔTsixmaternal X-chromosome in E6.5 extra-embryonic cells. (a) RNA FISH detection of Xist (white), Tsix (green), and Pgk1 (red) RNAs in E6.5 extra-embryonic cells. Nuclei are stained blue with 4′,6-diamidino-2-phenylindoledichloride (DAPI). Dashed boxes mark representative nuclei. Scale bar, 10 μm. (b) Quantification of Xist, Tsix and Pgk1 RNA expression patterns. Thexaxis of each graph represents the % nuclei in each class out of 100 total nuclei counted per genotype (fromn≥3 embryos per genotype). Diagrams along theyaxis depict all observed expression patterns. +, RNA expression detected from a single X-chromosome; ++, RNA expression detected from both X-chromosomes; −, absence of RNA detection. Pairwise comparisons of the frequency of individual gene expression patterns between WT andXΔTsix-mutant embryos were performed using Fisher’s exact test. *0.001<P<0.01; **P≤0.001. Extra-embryonic cells show significantly increased level of inactivation of theXΔTsixX-chromosome (P=0.0003 for males;P=3.5 × 10−5for females). (c) RT–PCR detection of Xist and Tsix RNAs in extra-embryonic tissues from individual E6.5 embryos. Results from three individual embryos of each genotype are shown. M, marker; NTC, no template control; +, RT; −, no RT control lane. (d) Sanger sequencing chromatograms of Xist RT–PCR products. Highlights mark a single nucleotide polymorphism that differs between the maternalXLabandXΔTsixalleles and the paternalXJF1allele.XLabXJF1females express Xist only from the paternally inherited X-chromosome (Xp), whileXΔTsixXJF1females express Xist biallelically in extra-embryonic tissues.XΔTsixYembryos variably express Xist from the maternally inherited X-chromosome. Figure 2: Xist induction from the X ΔTsix maternal X-chromosome in E6.5 extra-embryonic cells. ( a ) RNA FISH detection of Xist (white), Tsix (green), and Pgk1 (red) RNAs in E6.5 extra-embryonic cells. Nuclei are stained blue with 4′,6-diamidino-2-phenylindoledichloride (DAPI). Dashed boxes mark representative nuclei. Scale bar, 10 μm. ( b ) Quantification of Xist, Tsix and Pgk1 RNA expression patterns. The x axis of each graph represents the % nuclei in each class out of 100 total nuclei counted per genotype (from n ≥3 embryos per genotype). Diagrams along the y axis depict all observed expression patterns. +, RNA expression detected from a single X-chromosome; ++, RNA expression detected from both X-chromosomes; −, absence of RNA detection. Pairwise comparisons of the frequency of individual gene expression patterns between WT and X ΔTsix -mutant embryos were performed using Fisher’s exact test. *0.001< P <0.01; ** P ≤0.001. Extra-embryonic cells show significantly increased level of inactivation of the X ΔTsix X-chromosome ( P =0.0003 for males; P =3.5 × 10 −5 for females). ( c ) RT–PCR detection of Xist and Tsix RNAs in extra-embryonic tissues from individual E6.5 embryos. Results from three individual embryos of each genotype are shown. M, marker; NTC, no template control; +, RT; −, no RT control lane. ( d ) Sanger sequencing chromatograms of Xist RT–PCR products. Highlights mark a single nucleotide polymorphism that differs between the maternal X Lab and X ΔTsix alleles and the paternal X JF1 allele. X Lab X JF1 females express Xist only from the paternally inherited X-chromosome (Xp), while X ΔTsix X JF1 females express Xist biallelically in extra-embryonic tissues. X ΔTsix Y embryos variably express Xist from the maternally inherited X-chromosome. Full size image Differentiation-dependent function of Tsix in TS cells Whole-mount RNA FISH stains of Tsix-mutant E6.5 embryos suggested that ectopic Xist induction primarily characterized the trophectoderm-derived extra-embryonic ectoderm or its differentiated derivatives ( Supplementary Fig. 2a–d , Supplementary Movies 1–4 ). To further examine the role of Tsix in imprinted X-inactivation, we generated X Lab X JF1 , X ΔTsix X JF1 , X Lab Y and X ΔTsix Y trophoblast stem (TS) cells. TS cells arise from trophectoderm cells of the early embryo, and provide an in vitro model of imprinted X-inactivation [13] , [43] , [44] . Strand-specific RNA FISH analysis of the TS cells showed that Xist RNA is expressed from and coats a single X-chromosome in undifferentiated WT and X ΔTsix -mutant female TS cells, and is not expressed in male TS cells of either genotype ( Fig. 3a ). We confirmed that Xist RNA is restricted to female cells despite the absence of Tsix by allele-specific RT–PCR ( Fig. 3b ). These data not only reinforce the conclusion from embryos that X-inactivation is unperturbed in the absence of Tsix transcription from the maternal X-chromosome in trophectoderm cells, but also demonstrate that Tsix is not required to stably maintain Xist repression in undifferentiated TS cells in culture. 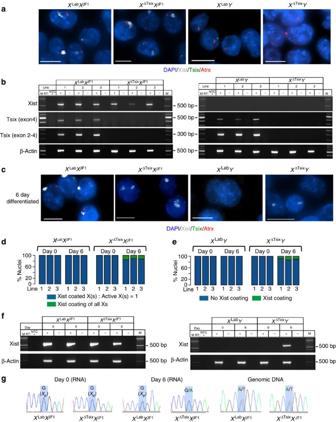Figure 3: TheXΔTsixmaternal X-chromosome displays ectopic Xist induction only upon differentiation in TS cells. (a) RNA FISH detection of Xist (white), Tsix (green) and Atrx (red) RNAs in representative TS cell lines. Nuclei are stained blue with 4′,6-diamidino-2-phenylindoledichloride (DAPI). Scale bar, 10 μm. Three cell lines of each genotype were analysed. (b) RT–PCR detection of Xist, Tsix (two different amplicons), and control β-actin RNAs in WT and Tsix-mutant TS cells. Three TS cell lines of each genotype were analysed. M, marker; NTC, no template control; +, RT; −, no RT control lane. (c) RNA FISH detection of Xist (white), Tsix (green) and Atrx (red) RNAs in 6-day (d6) differentiated TS cell lines. Three cell lines of each genotype were analysed. Scale bar, 10 μm. (d) Quantification of Xist induction from theXΔTsixX-chromosome in females. Aberrant Xist RNA coating (defined as two Xist RNA coats in a diploid cell or Xist coating of all X-chromosomes in polyploid giant cells) is observed in mutant but not WT d6-differentiated TS cells. For giant cells, the number of X-chromosomes was identified based on distinct Xist and Atrx RNA FISH signals.n=100 nuclei counted for each cell line per day of differentiation. (e) Quantification of Xist induction from theXΔTsixX-chromosome in males. Aberrant Xist RNA coating is observed in mutant but not WT d6 differentiated TS cells.n=100 nuclei counted for each cell line per day of differentiation. (f) RT–PCR detection of Xist and control β-actin RNA in undifferentiated (d0) and d6 differentiated WT and Tsix-mutant TS cells. A single representative TS cell line from each genotype is shown. M, marker; NTC, no template control; +, RT; −, no RT control lane. (g) Sanger sequencing chromatograms of representativeXLabXJF1andXΔTsixXJF1Xist RT–PCR products (RNA) and an Xist genomic DNA amplicon (gDNA) within exon 1. Highlights mark a single nucleotide polymorphism that differs between the maternalXLab/XΔTsixalleles and the paternalXJF1Xist allele. Figure 3: The X ΔTsix maternal X-chromosome displays ectopic Xist induction only upon differentiation in TS cells. ( a ) RNA FISH detection of Xist (white), Tsix (green) and Atrx (red) RNAs in representative TS cell lines. Nuclei are stained blue with 4′,6-diamidino-2-phenylindoledichloride (DAPI). Scale bar, 10 μm. Three cell lines of each genotype were analysed. ( b ) RT–PCR detection of Xist, Tsix (two different amplicons), and control β-actin RNAs in WT and Tsix-mutant TS cells. Three TS cell lines of each genotype were analysed. M, marker; NTC, no template control; +, RT; −, no RT control lane. ( c ) RNA FISH detection of Xist (white), Tsix (green) and Atrx (red) RNAs in 6-day (d6) differentiated TS cell lines. Three cell lines of each genotype were analysed. Scale bar, 10 μm. ( d ) Quantification of Xist induction from the X ΔTsix X-chromosome in females. Aberrant Xist RNA coating (defined as two Xist RNA coats in a diploid cell or Xist coating of all X-chromosomes in polyploid giant cells) is observed in mutant but not WT d6-differentiated TS cells. For giant cells, the number of X-chromosomes was identified based on distinct Xist and Atrx RNA FISH signals. n =100 nuclei counted for each cell line per day of differentiation. ( e ) Quantification of Xist induction from the X ΔTsix X-chromosome in males. Aberrant Xist RNA coating is observed in mutant but not WT d6 differentiated TS cells. n =100 nuclei counted for each cell line per day of differentiation. ( f ) RT–PCR detection of Xist and control β-actin RNA in undifferentiated (d0) and d6 differentiated WT and Tsix-mutant TS cells. A single representative TS cell line from each genotype is shown. M, marker; NTC, no template control; +, RT; −, no RT control lane. ( g ) Sanger sequencing chromatograms of representative X Lab X JF1 and X ΔTsix X JF1 Xist RT–PCR products (RNA) and an Xist genomic DNA amplicon (gDNA) within exon 1. Highlights mark a single nucleotide polymorphism that differs between the maternal X Lab / X ΔTsix alleles and the paternal X JF1 Xist allele. Full size image To reconcile why the extra-embryonic ectoderm in X ΔTsix X JF1 and X ΔTsix Y post-implantation embryos but not TS cells displayed ectopic Xist expression and X-inactivation, we hypothesized that Tsix is required in a differentiation-dependent manner, rather than a temporally specific manner, in the trophectoderm lineage. We therefore tested whether differentiation of X ΔTsix X JF1 and X ΔTsix Y TS cells would cause Xist induction from the Tsix-mutant X-chromosome. TS cell differentiation indeed led to ectopic Xist induction from the Tsix-mutant but not the WT maternal X-chromosome in both male and female cells by RNA FISH ( Fig. 3c–e ). We confirmed ectopic Xist induction from the maternal X ΔTsix in differentiated TS cells by allele-specific RT–PCR followed by Sanger sequencing ( Fig. 3f,g ). Next, we characterized when during differentiation TS cells induce Xist from the X ΔTsix . Only cells devoid of CDX2, a marker of trophoblast progenitor cells, displayed ectopic Xist induction ( Fig. 4a–d ). Moreover, Xist induction from the maternal X ΔTsix coincided with a failure of the mutant TS cells to differentiate to completion. Whereas WT TS cells of both sexes are able to terminally differentiate into trophoblast giant cells, X ΔTsix X JF1 and X ΔTsix Y TS cells displayed a significant reduction in the percentage of giant cells ( Fig. 4e,f ). Together, these results demonstrate that Tsix prevents Xist induction from the maternal X-chromosome during the differentiation of trophectodermal progenitor cells. Ectopic Xist induction and the ensuing inactivation of both Xs in females or of a single X in males results in a paucity of X-linked gene expression, which in turn is expected to cause reduced or stalled cell proliferation and prevent terminal differentiation. A block in TS cell differentiation is also consistent with the variable ectopic Xist induction and X-inactivation in the trophectoderm lineage of X ΔTsix X JF1 and X ΔTsix Y post-implantation embryos ( Fig. 2 , Supplementary Fig. 2 , Supplementary Movies 1–4 ). 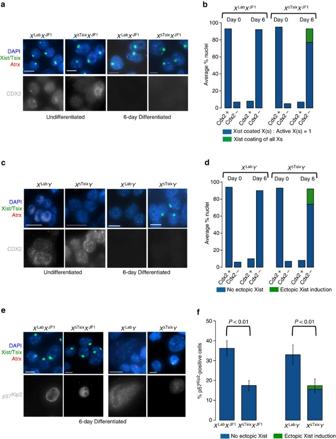Figure 4: Characterization of differentiation-dependent Xist RNA induction from theXΔTsixmaternal X-chromosome. (a) RNA FISH detection of Xist, Tsix, and the X-linked gene Atrx in undifferentiated and 6-day (d6) differentiated TS cells. IF staining of the same cells detects CDX2, a marker of undifferentiated trohoectodermal cells. Scale bar, 10 μm. (b) Quantification of Xist induction in CDX2 positive and negative in undifferentiated and differentiated female TS cells. One hundred nuclei were counted per cell line at each time point (n=3 cell lines per genotype). No aberrant Xist induction is observed from theXΔTsixin undifferentiated cells. In d6-differentiatedXΔTsixXJF1TS cells, ectopic Xist induction is restricted to cells that lack CDX2 staining. A subset of differentiated nuclei shows both multiple Xist-coated inactive X-chromosomes and multiple active X-chromosomes, due to endoreduplication. (c) IF/RNA FISH analysis of male TS cells, as in (a) scale bar, 10 μm. (d) Quantification of Xist induction in undifferentiated and d6-differentiated male TS cells. One hundred nuclei were counted per cell line at each time point (n=3 cell lines per genotype). (e) IF/RNA FISH detection of Xist, Tsix and the X-linked gene Atrx, in differentiated TS cells. p57Kip2, a marker of trophoblast giant cells, is detected in the same cells by IF. Scale bar, 10 μm. (f) Quantification p57Kip2-positive cells and aberrant Xist induction in the TS cells. One hundred nuclei were counted per cell line (n=3 cell lines per genotype).XΔTsixXJF1andXΔTsixYTS cells show significantly reduced levels of p57Kip2staining, suggesting failure of these genotypes to terminally differentiate. Error bars, s.d. Figure 4: Characterization of differentiation-dependent Xist RNA induction from the X ΔTsix maternal X-chromosome. ( a ) RNA FISH detection of Xist, Tsix, and the X-linked gene Atrx in undifferentiated and 6-day (d6) differentiated TS cells. IF staining of the same cells detects CDX2, a marker of undifferentiated trohoectodermal cells. Scale bar, 10 μm. ( b ) Quantification of Xist induction in CDX2 positive and negative in undifferentiated and differentiated female TS cells. One hundred nuclei were counted per cell line at each time point ( n =3 cell lines per genotype). No aberrant Xist induction is observed from the X ΔTsix in undifferentiated cells. In d6-differentiated X ΔTsix X JF1 TS cells, ectopic Xist induction is restricted to cells that lack CDX2 staining. A subset of differentiated nuclei shows both multiple Xist-coated inactive X-chromosomes and multiple active X-chromosomes, due to endoreduplication. ( c ) IF/RNA FISH analysis of male TS cells, as in ( a ) scale bar, 10 μm. ( d ) Quantification of Xist induction in undifferentiated and d6-differentiated male TS cells. One hundred nuclei were counted per cell line at each time point ( n =3 cell lines per genotype). ( e ) IF/RNA FISH detection of Xist, Tsix and the X-linked gene Atrx, in differentiated TS cells. p57 Kip2 , a marker of trophoblast giant cells, is detected in the same cells by IF. Scale bar, 10 μm. ( f ) Quantification p57 Kip2 -positive cells and aberrant Xist induction in the TS cells. One hundred nuclei were counted per cell line ( n =3 cell lines per genotype). X ΔTsix X JF1 and X ΔTsix Y TS cells show significantly reduced levels of p57 Kip2 staining, suggesting failure of these genotypes to terminally differentiate. Error bars, s.d. Full size image In addition to TS cells, XEN cells undergo imprinted X-inactivation of the paternal X-chromosome [43] , [45] . XEN cells are derived from the primitive endoderm layer of blastocysts that generates the extra-embryonic yolk sac in later-stage embryos. To test whether Tsix-mutant XEN cells can stably undergo imprinted X-inactivation, we derived X Lab X JF1 , X ΔTsix X JF1 , X Lab Y and X ΔTsix Y XEN cells. By both RNA FISH and allele-specific RT–PCR, we found that, just like in TS cells, XEN cells can stably repress Xist from the maternal X-chromosome independently of Tsix ( Fig. 5 ). 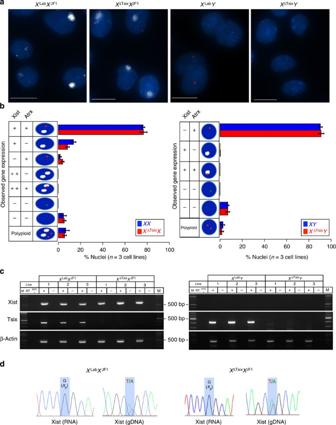Figure 5: Lack of Xist induction from theXΔTsixmaternal X-chromosome in cultured extra-embryonic endoderm (XEN) cells. (a) RNA FISH detection of Xist (white), Tsix (green) and Atrx (red) RNAs in representative XEN cell lines. Nuclei are stained blue with 4′,6-diamidino-2-phenylindoledichloride (DAPI). Three cell lines of each genotype were analysed. Scale bar, 10 μm. (b) Quantification of Xist RNA coating and X-linked gene expression in the XEN cells. Thexaxis of each graph represents average % nuclei in each class from 100 cells counted per cell line (n=3 cell lines per genotype). Diagrams along theyaxis depict all observed expression patterns. +, RNA expression detected from a single X-chromosome; + +, RNA expression detected from both X-chromosomes; −, absence of RNA detection. A subset of tetraploid XEN nuclei shows two Xist-coated inactive X-chromosomes and two active X-chromosomes, due to endoreduplication45. Gene expression patterns do not differ significantly between WT and Tsix-mutant XEN cells (Fisher’s exact test). Error bars, s.d. (c) RT–PCR detection of Xist, Tsix and control β-actin RNAs in three individual XEN cell lines of each genotype. M, marker; NTC, no template control; +, reaction with reverse transcriptase (RT); −, no RT control lane. (d) Sanger sequencing chromatograms of representativeXLabXJF1andXΔTsixXJF1RT–PCR products spanning Xist exons 1–4 (RNA), and an Xist genomic DNA amplicon (gDNA) within exon 1. Highlights mark a single nucleotide polymorphism that differs between the maternalXLab/XΔTsixalleles and the paternalXJF1allele. Figure 5: Lack of Xist induction from the X ΔTsix maternal X-chromosome in cultured extra-embryonic endoderm (XEN) cells. ( a ) RNA FISH detection of Xist (white), Tsix (green) and Atrx (red) RNAs in representative XEN cell lines. Nuclei are stained blue with 4′,6-diamidino-2-phenylindoledichloride (DAPI). Three cell lines of each genotype were analysed. Scale bar, 10 μm. ( b ) Quantification of Xist RNA coating and X-linked gene expression in the XEN cells. The x axis of each graph represents average % nuclei in each class from 100 cells counted per cell line ( n =3 cell lines per genotype). Diagrams along the y axis depict all observed expression patterns. +, RNA expression detected from a single X-chromosome; + +, RNA expression detected from both X-chromosomes; −, absence of RNA detection. A subset of tetraploid XEN nuclei shows two Xist-coated inactive X-chromosomes and two active X-chromosomes, due to endoreduplication [45] . Gene expression patterns do not differ significantly between WT and Tsix-mutant XEN cells (Fisher’s exact test). Error bars, s.d. ( c ) RT–PCR detection of Xist, Tsix and control β-actin RNAs in three individual XEN cell lines of each genotype. M, marker; NTC, no template control; +, reaction with reverse transcriptase (RT); −, no RT control lane. ( d ) Sanger sequencing chromatograms of representative X Lab X JF1 and X ΔTsix X JF1 RT–PCR products spanning Xist exons 1–4 (RNA), and an Xist genomic DNA amplicon (gDNA) within exon 1. Highlights mark a single nucleotide polymorphism that differs between the maternal X Lab / X ΔTsix alleles and the paternal X JF1 allele. Full size image Disassociation of H3-K27me3 enrichment and X-inactivation Xist RNA coating is postulated to lead to X-inactivation in cis [8] , [46] , [47] . We noticed, however, that in 5% of the E6.5 X ΔTsix X extra-embryonic cells Xist RNA coated both X-chromosomes, but one Xist-coated X-chromosome remained active, as indicated by expression of Pgk1 from one of the two Xs in these cells ( Fig. 2a,b ). In E6.5 X ΔTsix Y extra-embryonic nuclei, 17% of cells displayed both ectopic Xist RNA coating and Pgk1 expression from the single X-chromosome ( Fig. 2a,b ). To determine whether Pgk1 expression from the ectopically Xist RNA-coated X-chromosome agreed with expression of other X-linked genes subject to X-inactivation, we performed pairwise comparisons of expression of Pgk1 with Atrx and Atrx with Rnf12 ( Supplementary Fig. 3 ). We observed a high level of concordant expression of both sets of X-linked genes, leading to the conclusion that the ectopically Xist RNA-coated X-chromosome remained transcriptionally active in a subset of nuclei. To investigate the uncoupling of Xist RNA coating and X-linked gene silencing, we tested whether ectopic Xist RNA expression and coating led to the functional enrichment of the Polycomb group proteins on that X-chromosome. Xist RNA is thought to induce X-inactivation via the recruitment of protein complexes, most notably the Polycomb repressive complex 2 (PRC2), that inhibit transcription on the inactive-X [10] , [12] , [48] . PRC2 catalyses methylation of lysine at amino-acid position 27 in the tail of histone H3 (H3-K27me3), which is associated with transcriptional repression and is required for imprinted X-inactivation [10] , [12] , [43] , [49] . Moreover, both PRC2 components and H3-K27me3 accumulate on the inactive-X early during X-inactivation, suggesting an intimate role for PRC2 and H3-K27me3 in the formation of the inactive-X heterochromatin [10] , [12] . We therefore tested ectopic accumulation of PRC2-catalysed H3-K27me3 in E6.5 XX , X ΔTsix X , XY and X ΔTsix Y extra-embryonic cells. We found discordance between Xist RNA coating and H3-K27me3 accumulation; nuclei with ectopic Xist RNA coating in the Tsix-mutant cells did not always display H3-K27me3 enrichment ( Fig. 6a–c ). In cells with ectopic Xist RNA coating and concomitant H3-K27me3 accumulation, however, a substantial percentage (20% of female and 16% of male nuclei) harboured a transcriptionally competent X-chromosome, as reflected by Pgk1 expression ( Fig. 6b,c ). Together, these data demonstrate that Xist RNA induction often, but not always, leads to H3-K27me3 accumulation on the X ΔTsix maternal X-chromosome, and that X-inactivation does not necessarily follow. 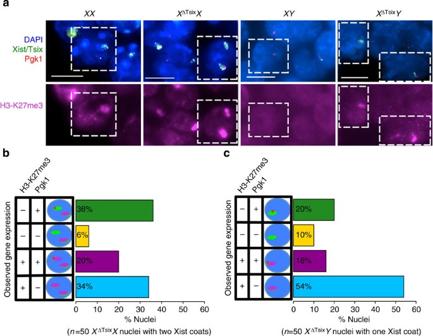Figure 6: Disassociation of Xist induction, H3-K27me3 enrichment and inactivation of theXΔTsixmaternal X-chromosome in E6.5 extra-embryonic cells. (a) RNA FISH detection of Xist, Tsix and Pgk1 RNAs coupled with IF detection of H3-K27me3 in extra-embryonic cells of E6.5 embryos. Dashed boxes mark representative nuclei. Scale bar, 10 μm. (b) Quantification of H3-K27me3 enrichment and Pgk1 expression in nuclei displaying Xist RNA coating of both X-chromosomes inXΔTsixXextra-embryonic cells (50 nuclei with Xist RNA coating of both X-chromosomes were analysed [n=5XΔTsixXembryos]). WTXXembryos show Xist RNA coating and enrichment of H3-K27me3 on a single X-chromosome (n=5 embryos). (c) Quantification of H3-K27me3 enrichment and Pgk1 expression in nuclei displaying Xist RNA coating of the X-chromosome inXΔTsixYextra-embryonic cells (50 nuclei with Xist RNA coating of the single X-chromosome [n=4XΔTsixYembryos] were analysed). WTXYcells show neither Xist RNA coating nor H3-K27me3 enrichment (n=4 embryos). Figure 6: Disassociation of Xist induction, H3-K27me3 enrichment and inactivation of the X ΔTsix maternal X-chromosome in E6.5 extra-embryonic cells. ( a ) RNA FISH detection of Xist, Tsix and Pgk1 RNAs coupled with IF detection of H3-K27me3 in extra-embryonic cells of E6.5 embryos. Dashed boxes mark representative nuclei. Scale bar, 10 μm. ( b ) Quantification of H3-K27me3 enrichment and Pgk1 expression in nuclei displaying Xist RNA coating of both X-chromosomes in X ΔTsix X extra-embryonic cells (50 nuclei with Xist RNA coating of both X-chromosomes were analysed [ n =5 X ΔTsix X embryos]). WT XX embryos show Xist RNA coating and enrichment of H3-K27me3 on a single X-chromosome ( n =5 embryos). ( c ) Quantification of H3-K27me3 enrichment and Pgk1 expression in nuclei displaying Xist RNA coating of the X-chromosome in X ΔTsix Y extra-embryonic cells (50 nuclei with Xist RNA coating of the single X-chromosome [ n =4 X ΔTsix Y embryos] were analysed). WT XY cells show neither Xist RNA coating nor H3-K27me3 enrichment ( n =4 embryos). Full size image Tsix is dispensable in X-chromosome reactivation In addition to preventing Xist RNA expression and X-inactivation, Tsix is also implicated in Xist repression in pluripotent ES cells, an in vitro analogue of the pluripotent epiblast precursor cells within the ICM of hatched blastocysts [37] , [38] , [39] . Loss of Xist RNA coating is a hallmark of the chromosome-wide epigenetic remodelling that accompanies reactivation of the inactive-X in epiblast precursors [29] , [30] , [33] . To test whether Tsix is required to repress Xist in the epiblast precursors, we isolated ICMs from XX and XX ΔTsix E4.0 embryos. In both XX and XX ΔTsix ICMs, we observed loss of Xist RNA coating and biallelic expression of Atrx , a gene subject to X-inactivation, indicating that reactivation of the paternal-X had occurred in spite of its lacking functional Tsix ( Fig. 7a–c ). We independently validated reactivation of the X ΔTsix paternal X-chromosome by allele-specific RT–PCR amplification of the X-linked genes Pdha1 , Rnf12 and Utx in E5.0 X JF1 X Lab and X JF1 X ΔTsix epiblasts ( Fig. 7d ). Whereas Pdha1 and Rnf12 are subject to X-inactivation, Utx escapes X-inactivation and serves as a control for the assay to gauge biallelic X-linked gene expression. If the paternal X-chromosome is reactivated, then transcription of all three genes should be apparent from both X-chromosomes. In agreement, all three genes displayed biallelic expression in both genotypes in E5.0 epiblasts. Based on these data, we conclude that the paternal X-chromosome is reactivated in pluripotent stem cells independently of Tsix. 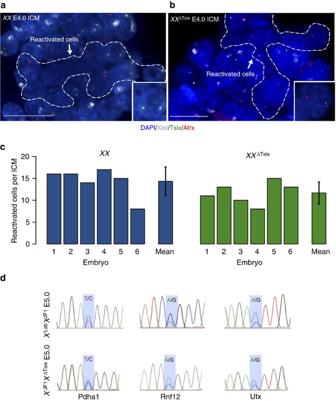Figure 7: Reactivation of the inactiveXΔTsixpaternal X-chromosome in the inner cell mass (ICM). RNA FISH detection of Xist (white), Tsix (green) and Atrx (red) RNAs in isolated (a)XXand (b)XXΔTsixE4.0 ICMs. Nuclei are stained blue with 4′,6-diamidino-2-phenylindoledichloride (DAPI). Insets show representative reactivated nuclei. Scale bar, 20 μm. (c) Quantification of the number of reactivated nuclei, as characterized by loss of Xist RNA coating and biallelic Atrx expression, in individual ICMs (n=6 ICMs per genotype). The mean number of reactivated cells per ICM does not differ significantly betweenXXandXXΔTsixICMs (P=0.23, two-tailedT-test). Error bars, s.d. (d) Allele-specific X-linked gene expression analysis in E5.0 epiblast cells. Representative chromatograms of sequenced cDNAs show biallelic expression of the X-linked genesPdha1, Rnf12,andUtx, regardless of genotype. Figure 7: Reactivation of the inactive X ΔTsix paternal X-chromosome in the inner cell mass (ICM). RNA FISH detection of Xist (white), Tsix (green) and Atrx (red) RNAs in isolated ( a ) XX and ( b ) XX ΔTsix E4.0 ICMs. Nuclei are stained blue with 4′,6-diamidino-2-phenylindoledichloride (DAPI). Insets show representative reactivated nuclei. Scale bar, 20 μm. ( c ) Quantification of the number of reactivated nuclei, as characterized by loss of Xist RNA coating and biallelic Atrx expression, in individual ICMs ( n =6 ICMs per genotype). The mean number of reactivated cells per ICM does not differ significantly between XX and XX ΔTsix ICMs ( P =0.23, two-tailed T -test). Error bars, s.d. ( d ) Allele-specific X-linked gene expression analysis in E5.0 epiblast cells. Representative chromatograms of sequenced cDNAs show biallelic expression of the X-linked genes Pdha1, Rnf12, and Utx , regardless of genotype. Full size image Tsix transcription across the Xist promoter is thought to inhibit Xist expression, and thereby prevent X-inactivation [17] , [18] . We show instead that Tsix is not required to repress Xist and prevent X-inactivation in the early embryo and in stem cells of the trophectoderm and primitive endoderm lineages. Earlier studies implicating Tsix in imprinted X-inactivation did not profile the onset of X-inactivation in Tsix-mutant preimplantation embryos or in TS and XEN cells [15] , [16] . We find that Tsix expression in cis is required to forestall inactivation of the maternal X-chromosome as the trophectoderm cells differentiate. By the post-implantation stage, the Tsix-mutant maternal X-chromosome displayed ectopic Xist RNA coating in 20 and 25%% of extra-embryonic cells isolated from E6.5 X ΔTsix X and X ΔTsix Y male and female embryos, respectively. The variable induction of Xist reflects a requirement for Tsix in differentiating but not undifferentiated trophoblast cells to prevent Xist induction and X-inactivation. Xist expression from and coating of the X ΔTsix maternal X-chromosome coincided with the enrichment of the histone modification H3-K27me3 on the mutant-X in many, but not all, X ΔTsix X (54%) and X ΔTsix Y (70%) extra-embryonic nuclei. Despite Xist RNA coating and H3-K27me3 accumulation, however, we unexpectedly found that 20% of the X ΔTsix maternal X-chromosomes in females and 16% in males did not undergo inactivation. This finding is consistent with and extends previous work showing that the recruitment of PRC2 and the catalysis of H3-K27me3 are insufficient to trigger gene silencing by ectopically integrated Xist transgenes or by a mutant Xist RNA expressed from the endogenous locus [10] , [12] , [50] . In these studies, however, the site of integration of the Xist transgene or the specific mutation in Xist cannot be excluded as the cause of defective silencing. We find that ectopic coating of the X-chromosome by an unmodified and endogenous Xist RNA followed by robust H3-K27me3 enrichment nevertheless results in active transcription of endogenous X-linked genes. Our work shows that the oocyte-derived imprint that prevents inactivation of the maternal X-chromosome in the early embryo does not act through Tsix RNA. We instead propose a model where the oocyte marks the maternal-X with chromosome-wide histone modifications, ensuring that genes along the maternal X-chromosome remain transcriptionally competent during early embryogenesis ( Fig. 8 ). This chromatin profile is sufficient to repress Xist during the initiation of imprinted X-inactivation in the early embryo independently of Tsix RNA. Tsix RNA is also not needed to maintain Xist repression in undifferentiated TS cells. During trophectodermal differentiation, by contrast, Tsix absence leads to Xist induction from and inactivation of the maternal-X. These data are consistent with previous findings that cellular differentiation can trigger X-inactivation defects, for example through large-scale chromatin changes that are inherent to differentiation [43] , [51] . The insufficiency of the germline-derived chromatin imprint to prevent inactivation of the maternal X-chromosome is also highlighted by the observations that the maternal-X in parthenogenetic embryos harbouring two maternal-Xs is subject to inactivation in extra-embryonic tissues of post-implantation embryos but not in preimplantation embryos [25] , [52] . We further propose that Tsix expression from the maternal X-chromosome is not directly programmed by the oocyte, but is simply a byproduct of the absence of Xist transcription from that chromosome. Indeed, Tsix RNA is induced when Xist expression is absent [52] , [53] . Tsix transcription then contributes to the chromatin structure at the Xist promoter region, and these Tsix-induced modifications may assume the Xist-inhibitory role in differentiating trophectodermal cells [17] , [18] . This mode of lncRNA function in epigenetic transcriptional regulation may also apply to other loci subject to imprinted, parent-of-origin-specific gene expression, where opposing sense–anti-sense lncRNA functions are invoked [54] . The reciprocal regulation by Tsix of Xist, in turn, is the cause of the Tsix-mutant maternal-Xs ectopically accumulating Xist RNA and H3-K27me3 in trophoblast cells. But, despite the enrichment of both Xist RNA and H3-K27me3, a significant percentage of X ΔTsix maternal X-chromosomes do not undergo inactivation. These findings are consistent with the hypothesis that factors in addition to or other than Xist RNA and H3-K27me3 contribute to the initiation of X-inactivation [21] , [43] , [55] . 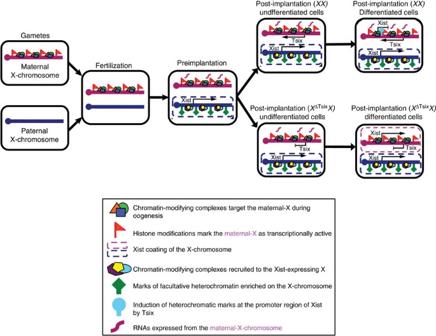Figure 8: A model for the role of Tsix in imprinted X-Inactivation. The maternal X-chromosome, but not the paternal-X, is marked by histone modifications during gametogenesis that are transmitted to the offspring upon fertilization. In the preimplantation embryo, these histone modifications prevent inactivation of the maternal-X, while the paternal X-chromosome is subject to inactivation. Xist is induced from the paternally derived X-chromosome in the preimplantation embryo, and helps recruit protein complexes that catalyse histone marks characteristic of facultative heterochromatin on the paternal-X. The oocyte-configured chromatin of the maternal-X, conversely, prevents Xist induction from the maternal X-chromosome during the initiation phase of X-inactivation (preimplantation) and does not require Tsix. The maternal-X then remains active during the maintenance phase of imprinted X-inactivation in undifferentiated extra-embryonic nuclei (post-implantation, undifferentiated cells), independently of Tsix expression. Tsix is induced from the maternal-X due to the absence of Xist expression from this X-chromosome. On differentiation, Tsix transcription across the Xist promoter region is required to induce heterochromatinization of the Xist promoter to keep Xist silenced in the extra-embryonic trophectodermal lineage. InXXdifferentiated extra-embryonic cells, the WT maternal-X remains transcriptionally competent while the paternal-X is maintained as transcriptionally inactive in imprinted X-inactivated cells. On differentiation ofXΔTsixXtrophectoderm cells, the Tsix-mutant maternal X-chromosome induces Xist. Figure 8: A model for the role of Tsix in imprinted X-Inactivation. The maternal X-chromosome, but not the paternal-X, is marked by histone modifications during gametogenesis that are transmitted to the offspring upon fertilization. In the preimplantation embryo, these histone modifications prevent inactivation of the maternal-X, while the paternal X-chromosome is subject to inactivation. Xist is induced from the paternally derived X-chromosome in the preimplantation embryo, and helps recruit protein complexes that catalyse histone marks characteristic of facultative heterochromatin on the paternal-X. The oocyte-configured chromatin of the maternal-X, conversely, prevents Xist induction from the maternal X-chromosome during the initiation phase of X-inactivation (preimplantation) and does not require Tsix. The maternal-X then remains active during the maintenance phase of imprinted X-inactivation in undifferentiated extra-embryonic nuclei (post-implantation, undifferentiated cells), independently of Tsix expression. Tsix is induced from the maternal-X due to the absence of Xist expression from this X-chromosome. On differentiation, Tsix transcription across the Xist promoter region is required to induce heterochromatinization of the Xist promoter to keep Xist silenced in the extra-embryonic trophectodermal lineage. In XX differentiated extra-embryonic cells, the WT maternal-X remains transcriptionally competent while the paternal-X is maintained as transcriptionally inactive in imprinted X-inactivated cells. On differentiation of X ΔTsix X trophectoderm cells, the Tsix-mutant maternal X-chromosome induces Xist. Full size image Our analysis additionally uncouples Tsix expression from the reactivation of the inactive paternal X-chromosome, a process that characterizes pluripotent epiblast precursor cells in the developing embryo [29] , [30] . X-reactivation is also a prominent epigenetic feature of pluripotent ES and iPSC cells [34] , [35] , [36] . Tsix induction from the inactive-X is posited to contribute to Xist repression and to the transcriptional equality of the two Xs in pluripotent cells [37] , [38] , [39] . We find, however, that despite Tsix absence, Xist RNA is repressed and the paternal X-chromosome is efficiently reactivated in epiblast precursor cells. In addition to by Tsix, Xist repression is postulated to occur via the pluripotency factors NANOG, OCT4, and SOX2, which are expressed in pluripotent epiblast progenitors and have been shown to bind within intron 1 of Xist in undifferentiated ES cells [37] , [39] , [56] , [57] . Thus, it is conceivable that these pluripotency factors may function to repress Xist and induce reactivation of the X ΔTsix paternal X-chromosome in the embryo. Countering this argument, however, Xist RNA upregulation and coating during random X-inactivation in the epiblast occurs despite high levels of NANOG, OCT4 and SOX2 expression, suggesting the involvement of additional factors in both Xist repression and X-reactivation [58] . Ethics statement This study was performed in strict accordance with the recommendations in the Guide for the Care and Use of Laboratory Animals of the National Institutes of Health. All animals were handled according to protocols approved by the University Committee on Use and Care of Animals (UCUCA) at the University of Michigan (Protocol #PRO00004007). Mice Mice harbouring the Tsix AA2Δ1.7 mutation were generated from targeted ES cells that were a kind gift of Takashi Sado and have been described elsewhere [16] , [55] . The mice recapitulate the published transmission frequency and phenotype [16] . The X-linked green fluorescent protein ( GFP ) transgenic strain is available via Jackson Labs (Tg(CAG-EGFP)D4Nagy/J) and have been described previously [21] , [43] , [55] , [59] . The M . molossinus JF1 strain was sourced from Jackson Laboratories (JF1/ms). Embryo dissections and processing E3.5–E4.0 embryos were flushed from the uterine limbs in 1 × phosphate-buffered saline (PBS) (Invitrogen, #14200075) containing 6% bovine serum albumin (BSA; Invitrogen, #15260037). Zona pellucidas surrounding E3.5 embryos were removed through incubation in cold acidic Tyrode’s Solution (Sigma, #T1788), immediately followed by neutralization through several transfers of cold M2 medium (Sigma, #M7167). GFP fluorescence conferred by the paternal transmission of the X-linked GFP transgene was used to distinguish female from male embryos, since only females inherit the paternal-X. Embryos were rinsed in 1X PBS with 6 mg ml −1 BSA, plated on gelatin-coated glass coverslips, excess solution was aspirated and the embryos air-dried for 15 min. After drying, embryos were permeabilized and fixed with 50 μl of 1X PBS containing 0.05% Tergitol (Sigma, #NP407) together with 1% paraformaldehyde for 10 min. Excess solution was tapped off, and coverslips were rinsed 3 times with 70% ethanol and stored in 70% ethanol at −20 °C before RNA FISH staining. For isolation of E5.0–E6.5 embryos, dissections were carried out in 1X PBS containing 6% BSA. Individual implantation sites were cut from the uterine limbs and decidua were removed with forceps. Embryos were dissected from the decidua, and the Reichert’s membranes surrounding post-implantation embryos were removed using fine forceps. For separation of extra-embryonic and epiblast portions of E6.5 embryos, fine forceps were used to physically bisect the embryos at the junction of the extra-embryonic ectoderm and epiblast. Immunofluorescence (IF) and/or RNA FISH staining were performed as described below. TS cells E3.5 embryos were flushed out from the uterus with MEMα (Invitrogen, #12561) with 10% fetal bovine serum (FBS; Invitrogen, #10439-024) and plated on mouse embryonic fibroblast cells in medium consisting of RPMI (Invitrogen, #21870076) with 20% FBS, 1 mM sodium pyruvate (Invitrogen, #11360-070), 100 μM β-mercaptoethanol (Sigma, #M7522), 2 mM L -glutamine (Invitrogen, #25030), 37.5 ng ml −1 FGF4 (R&D Systems, #235-F4-025), and 1.5 μg ml −1 heparin (Sigma, #H3149-10KU). Following five days of growth at 37 °C with 5% CO 2 , blastocyst outgrowths were dissociated with 0.05% trypsin (Invitrogen, #25300-054). Dissociated cells were plated on mouse embryonic fibroblasts and cultured at 37 °C with 5% CO 2 . RNA was collected from TS cells using Trizol (Invitrogen, #15596-018) and RT–PCR was performed as described below. For RNA FISH and/or IF, TS cells were split onto gelatin-coated glass coverslips and allowed to grow for 3–6 days. The cells were then permeabilized through sequential treatment with ice-cold cytoskeletal extraction buffer (CSK; 100 mM NaCl, 300 mM sucrose, 3 mM MgCl2 and 10 mM PIPES buffer, pH 6.8) for 30 s, ice-cold CSK buffer containing 0.4% Triton X-100 (Fisher Scientific, #EP151) for 30 s, followed twice with ice-cold CSK for 30 s each. After permeabilization, cells were fixed by incubation in 4% paraformaldehyde for 10 min. Cells were then rinsed 3 × in 70% ethanol and stored in 70% ethanol at −20 °C before IF and/or RNA FISH. For differentiation of TS cells, cells were split onto gelatinized dishes or coverslips and cultured for 6 days (d6) in media without FGF4 or heparin. On d6 of differentiation, RNA was harvested or cells were processed as described above for IF and RNA FISH. XEN cells E3.5 embryos were flushed from the uterus with MEMα with 10% FBS and plated on MEFs in XEN derivation medium consisting of MEMα with 50 μg/ml penicillin/streptomycin (Invitrogen, #15070063), 20% FBS, 1 mM sodium pyruvate, 100 μM β-mercaptoethanol, 2 mM L-glutamine, 100 μM nonessential amino acids (GIBCO, #11140–050), 1000 units/ml Leukemia Inhibitory Factor (LIF, Millipore #ESG1107). Following 6–8 days of growth at 37°C with 5% CO 2 , blastocyst outgrowths were dissociated with 0.05% trypsin. Dissociated cells were plated into individual wells of a 96-well dish containing MEFs and cultured at 37°C with 5% CO 2 . The cells were then split into a single well of a 4-well dish containing MEFs. After confluency, the cells were trypsinized and plated into a gelatinized well of a 6-well dish in XEN growth media (MEMα, 20% FBS, 1 mM sodium pyruvate, 100 μM β-mercaptoethanol, 2 mM L-glutamine, 100 μM nonessential amino acids). The cell lines were characterized as in ref. 43 [43] . RNA collection and processing for RNA FISH were performed as described for TS cells. RNA FISH Double-stranded RNA FISH (dsRNA FISH) probes were created by randomly priming DNA templates using BioPrime DNA Labeling System (Invitrogen, #18094011). Probes were labelled with Fluorescein-12-dUTP (Invitrogen), Cy3-dCTP (GE Healthcare, #PA53021), or Cy5-dCTP (GE Healthcare, #PA55031). Labelled probes for multiple genes were precipitated in a 3 M sodium acetate (Teknova, #S0298) solution along with 300 μg of yeast transfer RNA (Invitrogen, #15401-029), 15 μg of mouse COT-1 DNA (Invitrogen, #18440-016) and 150 μg of sheared, boiled salmon sperm DNA (Invitrogen, #15632-011). The solution was then spun at 15,000 r.p.m. for 20 min at 4 °C. The resulting pellet was washed in 70% ethanol, then washed in 100% ethanol, dried and resuspended in deionized formamide (ISC Bioexpress, #0606-500ML). The resuspended probe was denatured via incubation at 90 °C for 10 min followed by an immediate 5-min incubation on ice. A 2 × hybridization solution consisting of 4 × SSC, 20% Dextran sulphate (Millipore, #S4030), and 2.5 mg ml −1 purified BSA (New England Biolabs, #B9001S) was added to the denatured solution. The probe was then preannealed by incubation at 37 °C for 1 h to minimize probe hybridization to repetitive sequences. Probes were stored at −20 °C until use. Strand-specific RNA FISH (ssRNA FISH) probes were labelled with Fluorescein-12-UTP (Roche, #11427857910) or Cy3 CTP (GE Healthcare, # 25801086) using the Invitrogen MAXIscript Kit (Invitrogen, #AM-1324). Labelled probes were column purified (Roche, #11814427001). The labelled probes were then precipitated in 0.25 M ammonium acetate solution essentially as described above for dsRNA FISH probes, but without the addition of COT-1 DNA. Probes were resuspended as described for dsRNA FISH probes and stored at −20 without preannealing. Embryos, embryo fragments, TS cells, and XEN cells mounted on coverslips were dehydrated through 2 min incubations in 70, 85, 95 and 100% ethanol solutions and subsequently air-dried. The coverslips were then hybridized to the probe overnight in a humid chamber at 37 °C. The samples were then washed 3 × for 7 min each while shaking at 39 °C with 2XSSC/50% formamide, 2 × with 2 × SSC and 2 × with 1 × SSC. A 1:250,000 dilution of 4′,6-diamidino-2-phenylindoledichloride (Invitrogen, #D21490) was added to the third 2 × SSC wash. The embryos were then mounted in Vectashield (Vector Labs, #H-1200). A total of 64 E3.5 embryos (18 XX , 16 X ΔTsix X , 17 XY , and 13 X ΔTsix Y ) from eight litters were analysed by RNA FISH. For assessment of E4.0 embryos, 13 embryos from 2 litters were analysed by RNA FISH. Whole-mount RNA FISH E6.5 embryos were permeabilized through sequential transfers into ice-cold cytoskeletal extraction buffer (CSK;100 mM NaCl, 300 mM sucrose, 3 mM MgCl 2 and 10 mM PIPES buffer, pH 6.8) for 1 min, ice-cold CSK buffer containing 0.4% Triton X-100 (Fisher Scientific, #EP151) for 10 min, followed twice with ice-cold CSK for 1 min each. After permeabilization, the embryos were rinsed 3 × in 70% ethanol and stored in 70% ethanol at −20 °C before RNA FISH. Embryos were rehydrated by incubating in decreasing concentrations of ethanol diluted in 2 × SSC for 3 min each. Embryos were then placed in a droplet of 2 × SSC in a depression-well slide (Fisher Scientific, #S175201). Embryos were incubated in 10 μl of probe overnight in a depression-well slide (Fisher Scientific, #S175201) sealed with a glass coverslip in a humid chamber at 37 °C. Embryos were then rinsed with prewarmed (50 °C) 2 × SSC/50% deionized formamide (Amresco, #NC9473844) and washed with 50% formamide/2 × SSC solution 3 × for 15 min each at 50 °C, with periodic agitation via pipetting. Embryos were next washed with prewarmed 2 × SSC (50 °C) 3 × for 15 min each. In the first two 2 × SSC washes, 4′,6-diamidino-2-phenylindoledichloride (Invitrogen, #D21490) was included at a dilution of 1:200,000. Embryos were next washed in prewarmed 1 × SSC solution (50 °C) 2 × for 15 min each. After washing, embryos were processed through sequential incubations in PBS with 25, 50, 75 and 100% Vectashield (Vector Labs, #H-1000) and mounted in depression-well slides with Vectashield. PCR and allele-specific reverse trancriptase PCR Embryos and embryo fragments were lysed in 100 μl of lysis/binding buffer (Dynabeads mRNA DIRECT Micro Kit; Invitrogen, #610.21). Messenger RNA was isolated by following manufacturer’s instructions. SuperScript III One-Step RT–PCR Platinum Taq enzyme mixture (Invitrogen, #12574-035) was used to prepare and amplify the complimentary DNA (cDNA). Strand-specific reverse transcription of Xist was performed using the XR-9816 primer, which spans bp 9815-9775 of Xist (5′-CTCCACCTAGGGATCGTCAA-3′). For PCR amplification, the forward primer XF-9229, which spans bp 9229-9248 of Xist (5′-GACAACAATGGGAGCTGGTT-3′) was added upon completion of the RT reaction and before the PCR step. The Xist amplicon spans two introns, thus distinguishes any genomic DNA sequence amplification by size. Genomic PCR for the Xist locus was performed using the XR-721 primer, which spans 721–740 of Xist (5′-CGGGGCTTGGTGGATGGAAAT-3′), and XF-1083, which spans 1083-1064 of Xist (5′-GCACAACCCCGCAAATGCTA-3′). RT–PCR amplification of Tsix exon 4 in TS cells and E3.5 embryos was performed using the RT primer TR-4224, which spans base pairs 4224-4205 of Tsix (5′-TCGGATCCCACTACAGATGA-3′), and the forward PCR primer TF-3796, which spans base pairs 3796-3815 of Tsix (5′-CTAAGAGCACCTGGCTCCAC-3′). For E3.5 blastocysts, an additional round of nested PCR was performed to detect Tsix using TR-4224 and TF-3987, which spans base pairs 3987-4006 of Tsix (5′-TCCCAATTCTTGCAAACCTC-3′). RT–PCR for the Tsix amplicon spanning exons 2–4 was performed using the RT primer TR-732, which spans base pairs 732–713 of Tsix (5′-GGAGAGCGCATGCTTGCAAT-3′) and the forward PCR primer TF-350, which spans base pairs 350–369 of Tsix (5′-CCTGCAAGCGCTACACACTT-3′). RT–PCR for β-Actin was performed using the RT primer βA-R, which spans base pairs 673–655 of Actb (5′-GTAGCCACGCTCGGTCAGG-3′), and the forward primer βA-F, which spans base pairs 142–159 of Actb (5′-CGCGGGCGACGATGCTCC-3′). Amplified cDNAs were run on agarose gels and purified using the Clontech NucleoSpin Kit (Clontech, #740609). The purified cDNAs were then sequenced and sequencing traces were examined for single-SNPs characteristic of the M. musculus -derived X JF1 chromosome and the M. domesticus -derived WT X Lab and mutant X ΔTsix chromosomes. The SNP within the Xist amplicon localizes to bp 9399 of Xist . The M. domesticus -derived WT X Lab and mutant X ΔTsix SNP is an adenosine while the M. musculus- derived X JF1 SNP is a guanosine. The SNP within the Xist genomic PCR amplicon localizes to bp 804 of Xist . The M. domesticus -derived WT X Lab and mutant X ΔTsix SNP are thymidine while the M. musculus- derived X JF1 SNP is an adenosine. SNPs within X-linked genes Rnf12 (bp 860, NM_011276), Pdha1 (bp 969, NM_008810.2), and Utx (bp 1383, NM_009483.1) have been described previously [21] . RT and PCR primers for these genes have also been described previously [16] , [21] . Immunofluorescence Embryo fragments mounted on glass coverslips were washed 3 × in PBS for 3 min each while shaking. The fragments were then incubated in blocking buffer (0.5 mg ml BSA (New England Biolabs, #B9001S), 50 μg ml −1 yeast transfer RNA, 80 units ml −1 RNAseOUT (Invitrogen, #10777-019), and 0.2% Tween-20, in PBS) in a humid chamber for 30 min at 37 °C. The samples were next incubated with primary antibody, diluted in blocking buffer, for 1 h in the humid chamber at 37 °C. The H3-K27me3 (EMD Millipore, #ABE44) was used at 1:2,500 dilution in blocking buffer. The CDX2 antibody (BioGenex, #MU328A-UC) was used at a 1:75 dilution in blocking buffer. The p57 Kip2 antibody (Thermo Scientific, #RB-1637) was used at a 1:150 dilution in blocking buffer. Following three washes in PBS/0.2% Tween-20 for 3 min each while shaking, the embryos were incubated in blocking buffer for 5 min at 37 °C in the humid chamber. The embryos were then incubated in blocking buffer containing a 1:300 dilution of fluorescently conjugated secondary antibody (Alexa Fluor, Invitrogen) for 30 min in a humid chamber, followed by three washes in PBS/0.2% Tween-20 while shaking for 3 min each. The samples were then processed for RNA FISH as described above. Immunosurgery To isolate the ICM of E4.0 embryos, embryos were incubated in prewarmed rabbit anti-mouse serum (Rockland Immunochemicals, #110-4101) at a 1:5 dilution in M2 medium for 1 h in a humid chamber at 37 °C. After briefly rinsing in M2 medium, embryos were incubated in prewarmed guinea pig complement (Sigma, cat No. S1639) at a 1:5 dilution in M2 medium for 45 min to 1 h in a humid chamber at 37 °C. The embryos were then repeatedly pipetted using a finely pulled glass Pasteur pipette to remove trophectoderm cells. Isolated ICMs were treated with 0.05% trypsin for 10 min for mild dissociation, then incubated in M2 media with 10% FBS for 10 min to neutralize the trypsin. ICMs were then rinsed in 1 × PBS and permeabilized through sequential transfers into ice-cold CSK for 1 min, ice-cold CSK containing 0.4% Triton X-100 buffer for 5 min, followed twice with ice-cold CSK for 1 min each. ICMs were mounted on a glass coverslip coated with 1 × Denhardt’s solution in a small drop of ice-cold solution of 1 × PBS containing 1% paraformaldehyde and 20% CSK buffer. Excess solution was aspirated off and the coverslip air-dried for 15 min. The ICMs were then fixed in cold 3% paraformaldehyde for 10 min. After fixation, the coverslips were rinsed 3 × in 70% ethanol and stored in 70% ethanol at −20 °C before use. Microscopy Stained samples were imaged using a Nikon Eclipse TiE inverted microscope with a Photometrics CCD camera. The images were deconvolved and uniformly processed using NIS-Elements software. Statistics Comparisons between gene expression patterns were performed using a two-tailed Fisher’s exact test. P =0.01 was used as the cutoff for statistical significance. How to cite this article : Maclary, E. et al. Differentiation-dependent requirement of Tsix long non-coding RNA in imprinted X-chromosome inactivation. Nat. Commun. 5:4209 doi: 10.1038/ncomms5209 (2014).